SynDLP is a dynamin-like protein ofSynechocystissp. PCC 6803 with eukaryotic features Dynamin-like proteins are membrane remodeling GTPases with well-understood functions in eukaryotic cells. However, bacterial dynamin-like proteins are still poorly investigated. Syn DLP, the dynamin-like protein of the cyanobacterium Synechocystis sp. PCC 6803, forms ordered oligomers in solution. The 3.7 Å resolution cryo-EM structure of Syn DLP oligomers reveals the presence of oligomeric stalk interfaces typical for eukaryotic dynamin-like proteins. The bundle signaling element domain shows distinct features, such as an intramolecular disulfide bridge that affects the GTPase activity, or an expanded intermolecular interface with the GTPase domain. In addition to typical GD-GD contacts, such atypical GTPase domain interfaces might be a GTPase activity regulating tool in oligomerized Syn DLP. Furthermore, we show that Syn DLP interacts with and intercalates into membranes containing negatively charged thylakoid membrane lipids independent of nucleotides. The structural characteristics of Syn DLP oligomers suggest it to be the closest known bacterial ancestor of eukaryotic dynamin. Cells employ membrane remodeling proteins for diverse physiological processes, including endocytosis, exocytosis, membrane fusion and fission, and membrane repair [1] , [2] , [3] . Efficient membrane repair mechanisms are also indispensable for cells to cope with membrane damage, finally ensuring cell survival. Membrane remodeling is vital to maintain cellular compartmentalization by membrane-enclosed organelles in eukaryotes, as well as the maintenance of prokaryotic membrane systems. In fact, within the last decade, proteins have been identified in prokaryotes, which are involved in membrane repair and/or dynamics. Many of these proteins are homologs of proteins previously assumed to be eukaryotic inventions. Examples are the proteins FtsA, FtsZ and ZipA, which mediate membrane constriction during bacterial cytokinesis, and are homologous to the eukaryotic proteins tubulin, actin, and MAP-Tau [4] , [5] , [6] , [7] , [8] . Similarly, dynamins and dynamin-like proteins (DLPs) were originally assumed to be eukaryotic inventions until, in 1999, a bioinformatic study predicted the existence of bacterial DLPs (BDLPs) [9] . In eukaryotes, DLPs are involved in various membrane remodeling processes, such as endocytosis or fission and fusion of organelle membranes [10] , [11] , [12] , [13] , [14] , [15] , [16] , [17] . Unlike small (Ras-like) GTPases, DLPs are large mechanochemical GTPases with a molecular mass >60 kDa that use the energy gained via GTP hydrolysis for membrane binding and/or remodeling [18] . When bound, GTP is hydrolyzed, and cleavage of the γ-phosphate induces conformational changes leading to movements of conserved DLP domains relative to each other. The inorganic phosphate is then released, resulting in a GDP-bound DLP. Upon GDP dissociation, a new GTP can bind to the nucleotide-free enzyme to start a new cycle [19] . While DLP family members are typically not highly conserved on the sequence level, with the exception of the GTPase domain (GD), the resolved structures reveal a conserved modular arrangement of all DLPs: The globular GD at the protein’s N-terminus is typically followed by an α-helical bundle signaling element (BSE) or neck domain that connects the GD to an α-helical stalk or trunk domain. Most DLPs additionally have membrane interaction domains (MIDs) of varying designs [20] , [21] . The GD, the only structural element of DLPs that is conserved at the sequence level, is characterized by a low µM nucleotide binding-affinity plus a relatively high basal GTPase activity, at least when compared to other GTPases. E.g., Ras-like GTP-binding proteins require GTPase-activating proteins (GAPs) for nucleotide hydrolysis, whereas DLPs operate independently of GAPs [22] , [23] , [24] , [25] , [26] . Yet, the GTPase activity of DLPs typically increases when DLP monomers oligomerize, as the GTPase activity is regulated by intermolecular GD contacts leading to a head-to-head dimerization of adjacent GDs. E.g., dynamin dimers/tetramers show a basal GTPase activity of ~1 min −1 when free in solution. Yet, upon binding to membranes, dynamins oligomerize on the membrane surface, resulting in GTPase-activating GD contacts and release of auto-inhibitory GD-MID contacts [22] , [23] , [27] . This can finally increase the GTPase activity >100-fold [28] , [29] , [30] . Functionally, the majority of eukaryotic DLPs can be subdivided into either (i) membrane fission or (ii) membrane fusion DLPs [31] . Dynamin, the founder and namesake of the dynamin superfamily, is a fission DLP, involved in clathrin-mediated endocytosis [10] , [11] , [32] . Other fission DLPs, such as Drp1 and DRP3A, act on cell organelles, involving mitochondria and peroxisomes [12] , [13] . Conversely, fusion DLPs, such as mitofusin, OPA1 or atlastin, fuse the mitochondrial outer membrane, the mitochondrial inner membrane or the endoplasmic reticulum membrane, respectively [14] , [15] , [33] . The fusogenic DLP Fzl is involved in the remodeling of thylakoid membranes (TMs) in chloroplasts [16] , [17] , [34] . About two decades ago, a BDLP was characterized for the first time in the cyanobacterium Nostoc punctiforme ( Np BDLP) [35] . While the physiological functions of BDLPs are mostly enigmatic, a BDLP of Bacillus subtilis ( Bs DynA) has recently been shown to be involved in membrane stabilization and defense against phage infection [36] . For other BDLPs, several physiological functions were proposed, such as vesicle release or biogenesis ( Ec LeoA, Ms IniA) and crucial involvement in cytokinesis ( Sv DynA/B) [37] , [38] , [39] , [40] . As their eukaryotic counterparts, also BDLPs appear to be either involved in membrane fission or fusion, and, e.g., MsIniA has a membrane fission activity whereas Bs DynA and Cj -DLP1/2 are able to fuse membranes, at least in vitro [41] , [42] , [43] . Recently, a BDLP has also been identified in the genome of the cyanobacterium Synechocystis sp. PCC 6803 ( Syn DLP) [44] . In contrast to other prokaryotes, cyanobacteria typically contain an uncommon second, completely separated internal membrane system besides the cytoplasmic membrane, the TMs where the photosynthetic light reaction takes place. TMs have a rather unique lipid composition, with the two neutral galactolipids monogalactosyldiacylglycerol (MGDG) and digalactosyldiacylglycerol (DGDG) being the major membrane lipids, plus the negatively charged lipids sulfoquinovosyldiacylglycerol (SQDG) and the only phospholipid phosphatidylglycerol (PG) [45] , [46] . There are still many open questions concerning the biosynthesis of TMs, e.g., whether the TMs are completely assembled de novo or not [47] , [48] . Due to the photosynthetic light reaction, TMs are highly vulnerable to light stress and are continuously remodeled [49] , and thus, proteins mediating membrane remodeling and/or repair via membrane fusion and fission are required. As the involvement of DLPs in membrane dynamics and/or repair is well-established in eukaryotes, it is feasible to also assume involvement of Syn DLP in similar processes in Synechocystis sp. PCC 6803. Yet, currently Syn DLP solely is a predicted DLP and no information as to its structure and function are available. Here, we show that purified Syn DLP is a bona fide DLP that specifically interacts with negatively charged TM lipids. Furthermore, Syn DLP assembles into ordered high molecular mass oligomers. The structure of Syn DLP oligomers reveals oligomeric interfaces in the stalk domain typical for eukaryotic fission DLPs. Based on an analysis of an intramolecular disulfide bridge stabilizing the BSE and an assembly-impaired Syn DLP variant, we propose a GTPase activity-regulating function for the BSE domain. The interaction of Syn DLP with negatively charged lipid headgroups is nucleotide-independent. Cryo-EM structure of Syn DLP oligomers Recently, in a bioinformatic analysis, the orf slr0869 of the Synechocystis sp. PCC 6803 genome has been identified to encode a DLP ( Syn DLP) [44] . A sequence alignment and homology search revealed the presence of a GD with the typical GTP-binding motifs, including the G1-motif/P-loop, the G2-motif/switch I, the G3-motif/switch II and the G4-motif, all hallmarks of dynamin-like GTPases [18] , [20] , [21] . Syn DLP appears not to be essential in the cyanobacterium under standard growth conditions (Supplementary Fig. 1a ) albeit it is expressed in vivo (Supplementary Fig. 1b ). A typical sodium dodecyl sulfate polyacrylamide gel electrophoresis (SDS-PAGE) analysis of isolated, heterologously produced Syn DLP is shown in Supplementary Fig. 2 . Analytical size exclusion chromatography revealed that Syn DLP forms oligomers in solution, a feature typically observed when DLPs bind nucleotides or membranes (Fig. 1a ). Yet, in contrast to other BDLPs, Syn DLP forms high-molecular mass oligomers already in complete absence of an externally added membrane template and/or nucleotides. In a sedimentation assay, the addition of GTP or GDP led to only marginal changes in the sedimentation behavior of Syn DLP, indicating only a minor shift to larger structures in the presence of GTP and to smaller structures after GDP addition (Supplementary Fig. 3 ). When we visualized Syn DLP by cryo-EM using prepared plunge-frozen vitrified specimen, we observed short oligomeric filaments of bent half-moon shape (Fig. 1b ) with typical lengths of about 100 nm and a curvature radius of ~50 nm. Noteworthy, in contrast to biochemical assays, EM micrographs were acquired in the absence of NaCl, as the oligomeric filaments appeared longer and more defined under these conditions (Supplementary Fig. 4 ) and therefore more suitable for structural analysis. Class averages of these elongated oligomers revealed a width of 150 Å and a repeating unit every 60 Å along the oligomer (Fig. 1c ). Using a segmented single-particle analysis workflow (for details see Supplementary Fig. 5 ), we determined the structure of Syn DLP oligomers at an overall resolution of 3.7 Å (Fig. 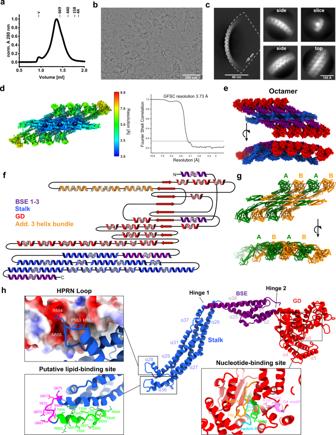Fig. 1: Cryo-EM structure of oligomericSynDLP. aAnalytical size exclusion chromatography ofSynDLP (black) revealed the formation of oligomeric structures that are larger than common standard proteins (standard proteins’ peak positions and molecular masses in kDa are indicated, v = void volume). Absorption values at 280 nm were normalized (0–1).bCryo-EM micrograph ofSynDLP oligomers. The data set of 8322 micrographs was measured one time (no independent replicates).cClass averages ofSynDLP oligomers with an enlarged oligomer side view including the curvature radius (left) and focused views of side, top, and slice view.dLocal resolution map and FSC curve (with auto-masking) of theSynDLP reconstruction.eModel of aSynDLP octamer with GD (red), BSE1-3 (purple) and stalk (blue).fSecondary structure topology plot ofSynDLP with additional α-helices of the enlargedSynDLP GD colored in orange.gModel of aSynDLP octamer highlighting the sequential arrangement of monomers within the oligomer. Alternating monomers are colored in green and orange, respectively.hModel of theSynDLP monomer, including structural features. GD, BSE and stalk are colored as in (e). Zoomed insets show the HPRN loop with the electrostatic surface of neighboring monomers, two putative lipid-binding sites at the tip of the stalk colored in magenta and green, respectively, and conserved motifs in the nucleotide-binding site of the GD: P-loop, switch I, switch II and G4 motif colored in green, orange, cyan and pink, respectively. 1d , Table 1 ). The local resolution varied from 3.0 to 3.5 Å at the stalk domain to 5.0 to 7.0 Å at the GD, presumably due to tighter contacts between the well-packed stalk domains and looser contacts between adjacent GDs. The last 19 residues at the C-terminus could not be resolved in the cryo-EM density, and thus, the final refined atomic model includes amino acids (aa) 1-793 of Syn DLP. Based on the determined cryo-EM map, we built a model of 8 Syn DLP monomers, which represents a smaller part of the segmented Syn DLP oligomer structure. When the determined octamer is extended, matching the observed dimensions of the 2D class averages, it will consist of ~40–50 monomers. The curvature radius of 50 nm of the Syn DLP oligomers is rather high compared to similar assemblies of other DLPs that typically assemble in the presence of membranes and/or nucleotides. Here, the curvature radius is usually in the range of 13 to 26 nm (reviewed here [20] ). However, other DLP assemblies also show a low curvature comparable to Syn DLP, e.g., Drp1 [50] . Fig. 1: Cryo-EM structure of oligomeric Syn DLP. a Analytical size exclusion chromatography of Syn DLP (black) revealed the formation of oligomeric structures that are larger than common standard proteins (standard proteins’ peak positions and molecular masses in kDa are indicated, v = void volume). Absorption values at 280 nm were normalized (0–1). b Cryo-EM micrograph of Syn DLP oligomers. The data set of 8322 micrographs was measured one time (no independent replicates). c Class averages of Syn DLP oligomers with an enlarged oligomer side view including the curvature radius (left) and focused views of side, top, and slice view. d Local resolution map and FSC curve (with auto-masking) of the Syn DLP reconstruction. e Model of a Syn DLP octamer with GD (red), BSE1-3 (purple) and stalk (blue). f Secondary structure topology plot of Syn DLP with additional α-helices of the enlarged Syn DLP GD colored in orange. g Model of a Syn DLP octamer highlighting the sequential arrangement of monomers within the oligomer. Alternating monomers are colored in green and orange, respectively. h Model of the Syn DLP monomer, including structural features. GD, BSE and stalk are colored as in ( e ). Zoomed insets show the HPRN loop with the electrostatic surface of neighboring monomers, two putative lipid-binding sites at the tip of the stalk colored in magenta and green, respectively, and conserved motifs in the nucleotide-binding site of the GD: P-loop, switch I, switch II and G4 motif colored in green, orange, cyan and pink, respectively. Full size image Table 1 Cryo-EM data collection and refinement statistics Full size table The Syn DLP structural model revealed a domain architecture typical for eukaryotic fission DLPs [27] , [50] (Fig. 1e–g ). The GD is flanked by parts of the BSE domain (N-terminally by BSE1, C-terminally by BSE2) followed by a stalk domain. The BSE3 domain part is located C-terminally to the stalk (Fig. 1f , Supplementary Fig. 6 ). The monomer model revealed a globular GD, linked via a flexible hinge region (hinge 2) to the mainly α-helical BSE domain, which is connected to an α-helical stalk via hinge 1 (Fig. 1h ). The oligomer structure showed a stalk backbone connected via a complex interaction network (Supplementary Fig. 7 ) from which the BSE domains and the GDs protrude laterally outwards (Fig. 1e ). The projected center of the stalk domains lies on a curve conferring the curvature of the Syn DLP oligomers. A loop consisting of an HPRN motif, which mediates critical contacts to neighboring monomers via electrostatic interactions (see below), as well as putative lipid-binding sites are located at the tip of the stalk (Fig. 1h ). Note that molecular details of the GD are more difficult to annotate due to the intermediate resolution of this part. Syn DLP is a potential bacterial ancestor of eukaryotic DLPs The Syn DLP monomer structure revealed typical DLP features (Fig. 1h ). The structure of Syn DLP oligomers resembles the assembly of eukaryotic fission DLPs via a complex network of interactions in the stalk domain, mainly mediated by three distinct interfaces (Supplementary Fig. 7b–d ). Interestingly, these interfaces are conserved in some eukaryotic DLPs [27] , [50] , [51] , yet, have not been reported in any prokaryotic DLP structure thus far (Supplementary Fig. 8a ). A surface conservation plot of Syn DLP revealed highly conserved residues in the nucleotide-binding pocket of the GD and laterally at the stalk (Fig. 2a , red-violet, Supplementary Fig. 9 ), which correspond to the conserved GD motifs and the oligomerization interfaces 2 and 3 (Fig. 1h , Supplementary Fig. 7c, d ). Structural analysis of isolated Syn DLP domains showed an increased size of the GD compared to other DLP GDs (Fig. 2b ). In fact, the Syn DLP GD is >100 aa larger than typical dynamin-like GDs as it contains additional loops and α-helices (Supplementary Fig. 10a ). In a structural alignment with eukaryotic and bacterial DLP representatives, the estimated root-mean-square deviation (RMSD) of Cα positions at 8.5–10.2 Å indicate a closer relation of Syn DLPs α-helices in the stalk domain to the eukaryotic DLP members Dyn3 and MxA as opposed to other bacterial members at >14 Å (Fig. 2c ), which is in line with the stalk-mediated assembly thus far observed solely in eukaryotic representatives (Supplementary Fig. 8a ). The close relation of Syn DLP to eukaryotic DLPs is further supported by structural alignments of isolated BSE domains (Supplementary Fig. 10b ). Taken together, Syn DLP is a prokaryotic DLP with an enlarged GD and shows structural features not observed in BDLPs before. Thus, Syn DLP is the closest known bacterial ancestor of a class of eukaryotic DLPs, such as dynamin or MxA. Fig. 2: Structural comparison of Syn DLP with other bacterial and eukaryotic DLP structures. a A surface conservation plot showed amino acids in the Syn DLP structure that are conserved in other DLP sequences. The surface conservation plot was produced using ConSurf [101] , [102] , [103] , [104] , [105] . The color key ranges from 1 (cyan, variable regions) to 9 (red-violet, conserved regions). The evaluation of single residues conservation in the primary sequence is shown in Supplementary Fig. 9 . The position of GD, BSE, and stalk are highlighted in the first side view. The oligomerization interfaces 1–3 are labeled in the second side view. b Structural side-by-side comparison of dynamin-like GDs from Syn DLP (gray) with a bacterial ( Np BDLP, PDB: 2J69, green) and a eukaryotic representative (Dyn3, PDB: 5A3F, red). The table summarizes the size of different GDs ( Syn DLP, Np BDLP (PDB: 2J69), Ms IniA (PDB: 6J73), Dyn3 (PDB: 5A3F), Drp1 (PDB: 5WP9) and MxA (PDB: 3SZR)). c Structural arrangement of α-helices in the stalk domains of Syn DLP (gray) and four other DLPs was compared by structural alignment of the domains leading to Cα-RMSD values larger than 10. The areas used for the structural alignments are highlighted in green ( Np BDLP), orange ( Ms IniA), red (Dyn3), blue (MxA) or magenta (Drp1) and the remaining structural elements not used for the alignment are colored in light gray. For details about the number of aligned residues, see Supplementary Fig. 10c . Full size image An intramolecular disulfide bridge in the BSE domain influences the Syn DLP GTPase activity The Syn DLP structure indicated the formation of an intramolecular disulfide bridge between C8 and C777 that covalently connects the BSE1 and BSE3 domains (Fig. 3a ). In fact, the migration behavior of Syn DLP in SDS-PAGE analysis changed depending on the DTT concentration (Fig. 3b ): at low DTT concentrations, i.e., when the disulfide bridge is established, Syn DLP ran at an increased apparent molecular mass whereas it ran at the predicted molecular mass in the presence of DTT. To study the structural impact of the intramolecular disulfide bridge, a Syn DLP variant was generated by mutating one of the involved cysteines (C777) to alanine. In the resulting protein ( Syn DLP C777A ) the formation of the disulfide bridge was prevented (Supplementary Fig. 2 ). When analyzed via size exclusion chromatography, Syn DLP C777A behaved like Syn DLP wt (Fig. 3c ), and thus, the C777A mutation apparently does not affect Syn DLP oligomer formation. In addition, the mutant protein seemed to be correctly folded at the secondary structure level as indicated by circular dichroism (CD) spectra of Syn DLP wt and Syn DLP C777A , which were identical at 20 °C (Fig. 3d ). Yet, the mutation affected the thermodynamic stability of Syn DLP. The thermal stability of Syn DLP wt and Syn DLP C777A was investigated by thermal denaturation of the proteins. Unfolding of the secondary structure was monitored via recording CD spectra in the far UV at increasing temperatures (Fig. 3e ). The spectra were dominated by minima at 208 and 222 nm, due to the high content of α-helices. While from the melting curve of Syn DLP wt (Fig. 3e , black) a T m, CD of 49.5 ± 0.3 °C was calculated, the T m, CD of the Syn DLP C777A variant (Fig. 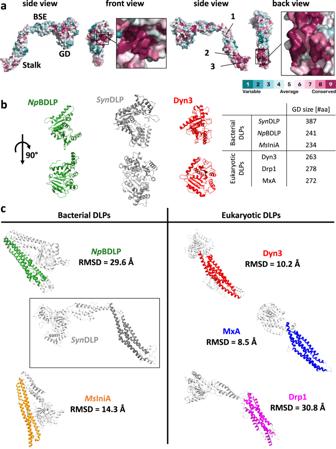Fig. 2: Structural comparison ofSynDLP with other bacterial and eukaryotic DLP structures. aA surface conservation plot showed amino acids in theSynDLP structure that are conserved in other DLP sequences. The surface conservation plot was produced using ConSurf101,102,103,104,105. The color key ranges from 1 (cyan, variable regions) to 9 (red-violet, conserved regions). The evaluation of single residues conservation in the primary sequence is shown in Supplementary Fig.9. The position of GD, BSE, and stalk are highlighted in the first side view. The oligomerization interfaces 1–3 are labeled in the second side view.bStructural side-by-side comparison of dynamin-like GDs fromSynDLP (gray) with a bacterial (NpBDLP, PDB: 2J69, green) and a eukaryotic representative (Dyn3, PDB: 5A3F, red). The table summarizes the size of different GDs (SynDLP,NpBDLP (PDB: 2J69),MsIniA (PDB: 6J73), Dyn3 (PDB: 5A3F), Drp1 (PDB: 5WP9) and MxA (PDB: 3SZR)).cStructural arrangement of α-helices in the stalk domains ofSynDLP (gray) and four other DLPs was compared by structural alignment of the domains leading to Cα-RMSD values larger than 10. The areas used for the structural alignments are highlighted in green (NpBDLP), orange (MsIniA), red (Dyn3), blue (MxA) or magenta (Drp1) and the remaining structural elements not used for the alignment are colored in light gray. For details about the number of aligned residues, see Supplementary Fig.10c. 3e , red) was determined to be 43.7 ± 0.3 °C (Table 2 ), showing that Syn DLP C777A is less stable than the wt. This observation was further elucidated via an ANS fluorescence thermal shift assay (FTSA), which monitors changes in the tertiary and quaternary structure of proteins and thus complements the CD measurements. The T m, ANS-FTSA was shifted by ~8 °C from 46.7 ± 0.1 °C to 39.0 ± 0.1 °C for the mutant (Fig. 3f , Table 2 ), which further confirmed the lowered thermodynamic stability of Syn DLP C777A compared to Syn DLP wt. Fig. 3: Structural stabilization and enhanced GTPase activity by an intramolecular disulfide bridge in the BSE domain. a Ribbon representation of a Syn DLP monomer. C8 and C777, forming an intramolecular disulfide bridge that connects BSE1 and BSE3, are highlighted in green. BSE1, which consists of two α-helices, BSE2 and BSE3 are colored purple, gray and magenta, respectively. GD colored in red, stalk in blue. b Syn DLP was incubated with different DTT concentrations (the final concentrations after adding SDS sample buffer are given). The amount of Syn DLP with an intact disulfide bridge depended on the DTT concentration (band with intact bridge at ~180 kDa, band with reduced cysteines at ~100 kDa). M = marker. Representative gel from two independent experiments with the same result. c Analytical size exclusion chromatography of Syn DLP C777A (red) compared to Syn DLP wt (black) revealed the formation of oligomeric structures for both proteins. A 280 values were normalized (0–1) for better comparison. d CD spectra of 1 µM Syn DLP wt (black) and Syn DLP C777A (red). Mean of three measurements is shown. For comparison, the spectra were normalized (θ value at 250 nm set to 0, minimum θ set to −1). e The thermal stability of Syn DLP (black) and Syn DLP C777A (red) was monitored using CD spectroscopy. The ellipticities at 222 nm were plotted against the temperature, normalized (0–1) and fitted with an adapted Boltzmann fit (Eq. ( 3 )). The fit curves are shown as lines. Mean of independent measurements ( n = 3) and error bars (S.D.) are shown. f Measured ANS-FTSA of Syn DLP wt (black) and Syn DLP C777A (red). ANS fluorescence intensities at 470 nm were plotted against the temperature and normalized (0–1) for better comparison. A temperature range capturing the transition phase was fitted with an adapted Boltzmann fit (Eq. ( 4 )). Fit curves are shown as lines. The mean of three independent experiments and error bars (S.D.) are displayed. g The GTPase activity of Syn DLP wt (black) and Syn DLP C777A (red) were measured in a continuous, regenerative, coupled assay. The mean and error bars (S.D.) of three independent experiments are shown. The data points were fitted using Eq. ( 2 ). Full size image Table 2 Transition temperatures of Syn DLP variants determined via CD spectroscopy and ANS-FTSA Full size table As DLPs catalyze the hydrolysis of GTP to GDP and P i , the GTPase activity of Syn DLP and Syn DLP C777A was determined next via a continuous, regenerative, coupled GTPase assay. Typically, the GTPase assay was performed with 0.5 µM protein, as Syn DLP showed a concentration-dependent GTPase activity at low protein concentrations yet reaching a plateau at protein concentrations >0.3 µM (Supplementary Fig. 11a ), and in the presence of the monovalent cations Na + and K + , which were shown to activate the GTP hydrolysis catalyzed by DLPs [22] . E.g., the omission of NaCl led to a clear decrease of the Syn DLPs GTPase activity (Supplementary Fig. 11b ). A mutation of a conserved residue in the P-loop (K61A) considerably reduced the GTPase activity, as previously observed for dynamin and other DLPs, which demonstrated a related GTPase mechanism (Supplementary Fig. 11c ). The GTPase activities of Syn DLP wt and C777A followed a typical Michaelis-Menten kinetic (Fig. 3g ), and consequently the data were fitted with a hyperbolic curve (Eq. ( 2 )). 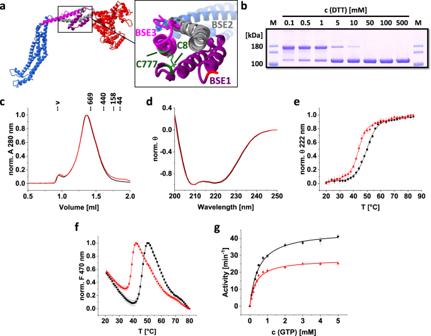Fig. 3: Structural stabilization and enhanced GTPase activity by an intramolecular disulfide bridge in the BSE domain. aRibbon representation of aSynDLP monomer. C8 and C777, forming an intramolecular disulfide bridge that connects BSE1 and BSE3, are highlighted in green. BSE1, which consists of two α-helices, BSE2 and BSE3 are colored purple, gray and magenta, respectively. GD colored in red, stalk in blue.bSynDLP was incubated with different DTT concentrations (the final concentrations after adding SDS sample buffer are given). The amount ofSynDLP with an intact disulfide bridge depended on the DTT concentration (band with intact bridge at ~180 kDa, band with reduced cysteines at ~100 kDa). M = marker. Representative gel from two independent experiments with the same result.cAnalytical size exclusion chromatography ofSynDLPC777A(red) compared toSynDLP wt (black) revealed the formation of oligomeric structures for both proteins. A280values were normalized (0–1) for better comparison.dCD spectra of 1 µMSynDLP wt (black) andSynDLPC777A(red). Mean of three measurements is shown. For comparison, the spectra were normalized (θ value at 250 nm set to 0, minimum θ set to −1).eThe thermal stability ofSynDLP (black) andSynDLPC777A(red) was monitored using CD spectroscopy. The ellipticities at 222 nm were plotted against the temperature, normalized (0–1) and fitted with an adapted Boltzmann fit (Eq. (3)). The fit curves are shown as lines. Mean of independent measurements (n= 3) and error bars (S.D.) are shown.fMeasured ANS-FTSA ofSynDLP wt (black) andSynDLPC777A(red). ANS fluorescence intensities at 470 nm were plotted against the temperature and normalized (0–1) for better comparison. A temperature range capturing the transition phase was fitted with an adapted Boltzmann fit (Eq. (4)). Fit curves are shown as lines. The mean of three independent experiments and error bars (S.D.) are displayed.gThe GTPase activity ofSynDLP wt (black) andSynDLPC777A(red) were measured in a continuous, regenerative, coupled assay. The mean and error bars (S.D.) of three independent experiments are shown. The data points were fitted using Eq. (2). The turnover rate (k cat ) and the Michaelis-Menten constant (K m ) were determined, as summarized in Table 3 . Apparently, with a k cat of 44.6 ± 1.0 min −1 Syn DLP had a relatively high basal GTPase activity (Fig. 3g , black). Yet, the turnover rate of the Syn DLP C777A mutant was significantly reduced by almost 40% compared to the wt (Fig. 3g , red, Table 3 ). Next, GTP binding affinities of Syn DLP wt and C777A were determined via fluorescence anisotropy measurements using the GTP analog Mant-GTP (Supplementary Fig. 12 ). Based on this assay, both proteins have similar nucleotide-binding affinities in the three-digit nanomolar range. As both proteins showed no residual (measurable) GTPase activity at 0 mM GTP (negative control without nucleotide; first data point in each curve) although a GTP regenerating system was added, we conclude that no significant amount of GTP/GDP has been co-purified with the proteins. This is supported by the low A 260 /A 280 ratio of 0.7 determined via absorption spectroscopy using purified Syn DLP, a value indicating that no nucleotides were bound. Table 3 Kinetic parameters describing the GTPase activity of Syn DLP variants Full size table Uncommon GD contacts enhance the Syn DLP GTPase activity In the Syn DLP oligomer structure we observed an expanded intermolecular GD-BSE1 interface (Fig. 1e , Supplementary Fig. 8b ). The role of the intermolecular GD-BSE1 interface in Syn DLP oligomers was addressed via analysis of an assembly-defective Syn DLP variant. Syn DLP oligomerizes via an intricate interaction network in the stalk domain by contacts of defined interfaces as already mentioned (Supplementary Fig. 7 ). As a general feature, structurally related DLPs form a stable dimer via interface 2. The basic dimeric unit can tetramerize or further oligomerize via interfaces 1 and 3. The latter is non-symmetric and mediates lateral contacts between parallelly oriented stalks. Following previous studies on diverse DLPs where oligomerization was disturbed by mutations, we replaced the residues 552 HPRN 555 in a highly conserved loop at the tip of the stalk domain that is part of oligomerization interface 3 (Fig. 1h , Supplementary Fig. 13a ) [52] , [53] , [54] , [55] , [56] by four alanines. The migration behavior of Syn DLP HPRN-AAAA on an SDS PAGE gel (Fig. 4a ) and the wt-like shape of the CD spectrum (Fig. 4b ) indicated proper secondary structure formation as well as the formation of the stabilizing disulfide bridge within the BSE of the mutated protein. Yet, analytical size exclusion chromatography of Syn DLP HPRN-AAAA revealed an apparent MW of ~174 kDa, indicating formation of dimers (Fig. 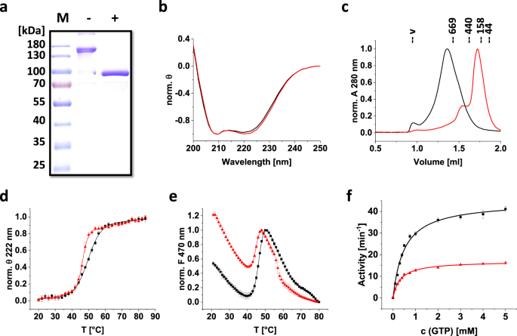Fig. 4: Biochemical analysis ofSynDLPHPRN-AAAA. aPurifiedSynDLPHPRN-AAAAwas analyzed via SDS-PAGE in the presence of 0.1 mM DTT (lane −) or 100 mM DTT (lane +). The calculated molecular mass of the protein is 93 kDa. The SDS-PAGE analysis revealed a single band at ~100 kDa (lane +) without showing further protein bands, thus the protein was ≥95% pure. M = marker. Representative gel of two independent experiments showing the same results.bCD spectra ofSynDLP wt (black) andSynDLPHPRN-AAAA(red). The mean of three measurements is shown. The spectra were normalized (θ value at 250 nm set to 0, minimum θ set to −1) for better comparison.cAnalytical size exclusion chromatography ofSynDLP wt (black) andSynDLPHPRN-AAAA(red). The elution peak positions of the standard proteins and the corresponding molecular masses are indicated (v = void volume). A280values were normalized (0–1) to better compare the chromatograms.dCD spectra ofSynDLP wt (black) andSynDLPHPRN-AAAA(red) were recorded at increasing temperatures. The ellipticities at 222 nm were plotted against the temperature, normalized (0–1) and fitted with an adapted Boltzmann fit (Eq. (3)). The fit curves are displayed as lines. Mean of three independent experiments and error bars (S.D.) are shown.eANS-FTSA measurements ofSynDLP wt (black) andSynDLPHPRN-AAAA(red). ANS fluorescence intensities at 470 nm were plotted against the temperature and normalized (minimum set to 0, main peak set to 1). The temperature range that captured the transition phase was fitted with an adapted Boltzmann fit (Eq. (4)). Fit curves are shown as lines. Error bars represent S.D.,n= 3 (mean of independent measurements).fGTPase activity of 0.5 µMSynDLP (black) orSynDLPHPRN-AAAA(red). Mean of independent experiments (n= 3) and error bars (S.D.) are shown. Data points were fitted using the Michaelis-Menten equation (Eq. (2)). The fit curves are displayed as lines. 4c , red), which was previously also observed for other DLPs carrying the equivalent mutations [52] , [53] , [56] . 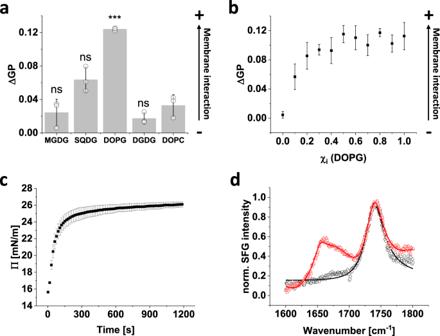Fig. 5: Membrane interaction ofSynDLP. aFluorescence spectroscopy using Laurdan as a fluorescent probe. LUVs were prepared with 50% DOPC and 50% of the indicated TM lipid (w/w) mixed with Laurdan at a 1:500 molar ratio. Laurdan fluorescence emission was measured after 30 min incubation ofSynDLP and LUVs and the ΔGP value was calculated from the spectra. Mean of three independent experiments (single measurements shown as circles) and error bars (S.D.) are shown. ns = not significant (P> 0.05), *P< 0.05, **P< 0.01, ***P< 0.001 based on a two-sided unpaired Student’s t-test. The ΔGP values of MGDG (P= 0.52), SQDG (P= 0.055), DOPG (P= 0.00028) or DGDG (P= 0.14) are compared to DOPC. Arrow indicates increasing membrane interaction.bLUVs were prepared with different DOPG/DOPC molar ratios (Laurdan added at a 1:500 molar ratio). Laurdan fluorescence spectra were recorded after 30 min and ΔGP values (black) were determined from the spectra. Mean of independent measurements (n= 4) and error bars (S.D.) are shown. Arrow indicates increasing membrane interaction.cProgression of the surface pressure (black) measured over time in parallel to the SFG intensity shown in (d). SFG spectroscopy of 0.5 µMSynDLP was carried out on a DMPG monolayer under reaction buffer conditions (without DTT).t= 0 s corresponds to the moment ofSynDLP addition. Mean of three independent measurements and error bars (S.D.) are shown.dThe SFG spectrum in the amide I region of the DMPG monolayer (black) and afterSynDLP addition and equilibration (red) is shown. A fit of the amide I band is displayed as a line. The mean of three independent measurements is shown. SFG intensity was normalized (0–1) for better comparison. The hampered oligomerization was also confirmed by cryo-EM micrographs (Supplementary Fig. 13b+c ). Thermal denaturation of Syn DLP and Syn DLP HPRN-AAAA was monitored via CD spectroscopy and ANS-FTSA to investigate the impact of oligomerization on the thermodynamic stability. With both methods, a slight decrease of the T m of Syn DLP HPRN-AAAA was observed, which indicated that oligomerization promotes the thermodynamic stability (Fig. 4d, e , Table 2 ). Compared to Syn DLP wt (Fig. 4e , black), the ANS-FTSA curve of Syn DLP HPRN-AAAA (Fig. 4e , red) indicated increased hydrophobic, ANS-accessible surface regions, visible as an increased starting F 470 nm value at 20 °C. Most likely, surface regions, which are not covered in the assembly-defective mutant protein, are now ANS accessible, leading to an increased initial ANS fluorescence emission. Fig. 4: Biochemical analysis of Syn DLP HPRN-AAAA . a Purified Syn DLP HPRN-AAAA was analyzed via SDS-PAGE in the presence of 0.1 mM DTT (lane −) or 100 mM DTT (lane +). The calculated molecular mass of the protein is 93 kDa. The SDS-PAGE analysis revealed a single band at ~100 kDa (lane +) without showing further protein bands, thus the protein was ≥95% pure. M = marker. Representative gel of two independent experiments showing the same results. b CD spectra of Syn DLP wt (black) and Syn DLP HPRN-AAAA (red). The mean of three measurements is shown. The spectra were normalized (θ value at 250 nm set to 0, minimum θ set to −1) for better comparison. c Analytical size exclusion chromatography of Syn DLP wt (black) and Syn DLP HPRN-AAAA (red). The elution peak positions of the standard proteins and the corresponding molecular masses are indicated (v = void volume). A 280 values were normalized (0–1) to better compare the chromatograms. d CD spectra of Syn DLP wt (black) and Syn DLP HPRN-AAAA (red) were recorded at increasing temperatures. The ellipticities at 222 nm were plotted against the temperature, normalized (0–1) and fitted with an adapted Boltzmann fit (Eq. ( 3 )). The fit curves are displayed as lines. Mean of three independent experiments and error bars (S.D.) are shown. e ANS-FTSA measurements of Syn DLP wt (black) and Syn DLP HPRN-AAAA (red). ANS fluorescence intensities at 470 nm were plotted against the temperature and normalized (minimum set to 0, main peak set to 1). The temperature range that captured the transition phase was fitted with an adapted Boltzmann fit (Eq. ( 4 )). Fit curves are shown as lines. Error bars represent S.D., n = 3 (mean of independent measurements). f GTPase activity of 0.5 µM Syn DLP (black) or Syn DLP HPRN-AAAA (red). Mean of independent experiments ( n = 3) and error bars (S.D.) are shown. Data points were fitted using the Michaelis-Menten equation (Eq. ( 2 )). The fit curves are displayed as lines. Full size image Next, the GTPase activity of Syn DLP HPRN-AAAA was measured to evaluate the impact Syn DLP oligomerization has on its GTP hydrolyzing activity. If Syn DLP HPRN-AAAA dimerization via oligomeric interface 2 is assumed (Supplementary Fig. 7 ), the assembly-defective protein is not expected to form the intermolecular GD contacts anymore that were observed in the Syn DLP wt oligomers. The activity of Syn DLP wt (black) and Syn DLP HPRN-AAAA (red) at different substrate concentrations is shown in Fig. 4f . As the wt, the activity of Syn DLP HPRN-AAAA followed a typical Michaelis-Menten kinetic. The fit with a hyperbolic curve revealed a k cat of 17.0 ± 0.2 min −1 for Syn DLP HPRN-AAAA (Table 3 ), and thus, the turnover rate was reduced by ~60% in case of the assembly-defective protein. The GTP binding affinity of the mutant appeared not to be significantly affected as indicated by a Mant-GTP binding assay (Supplementary Fig. 12 ). 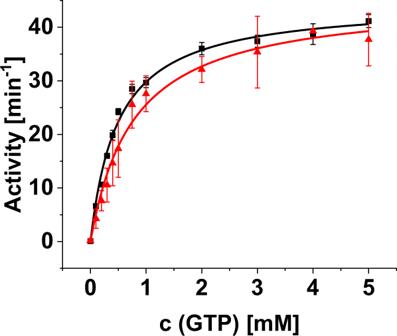Fig. 6: Lipid-stimulation of theSynDLP GTPase activity. SynDLP GTPase activities in the presence and absence of LUVs were determined in a continuous, regenerative, coupled assay. Comparison ofSynDLP under standard measurement conditions (black) and with 50 µM DOPG LUVs (dissolved in reaction buffer, extrusion to 100 nm) added with the assay components (red). Mean of independent experiments (n= 3) and error bars (S.D.) are shown. Data points were fitted using the Michaelis-Menten equation (Eq. (2)). Fit curves are shown as lines. 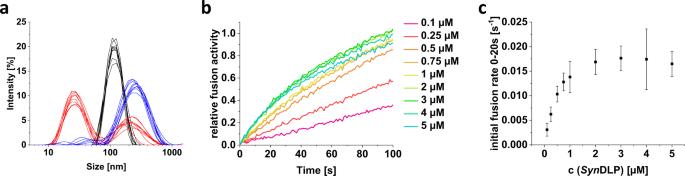Fig. 7: Membrane fusion activity ofSynDLP. aSize distribution of protein and LUVs was analyzed using DLS and relative intensities of the respective sizes are shown. MGDG/DOPG (60%/40%,w/w) LUVs (black),SynDLP (red) or a mixture of LUVs andSynDLP (blue) were incubated in reaction buffer and measured. From each condition the size distribution of three independent measurements (+ three technical replicates of each measurement) are shown.bFusion of MGDG/DOPG (60%/40%,w/w) LUVs was measured in the presence of increasingSynDLP concentrations using a FRET-based fusion assay. Curves showing the donor fluorescence over the first 100 s after mixing LUVs with protein. The relative fusion activities were calculated as described in the methods section. The curves represent the mean of three independent measurements. The whole measurement as well as the positive control containing 2 µM of the fusogenic protein IM30 are shown in Supplementary Fig.18.cInitial fusion rates (black) were calculated from the curves in (b) defined as the slope of a linear regression of the first 20 s. Mean of independent measurements (n= 3) and error bars (S.D.) are shown. Syn DLP interacts with negatively charged TM lipids While Syn DLP is per se a soluble protein, membrane interaction of Syn DLP is a prerequisite for catalyzing membrane dynamics. Thus, the membrane interaction propensity of Syn DLP was next investigated. First, the membrane interaction of Syn DLP with the main TM lipid species MGDG, SQDG, DGDG and PG was tested via fluorescence spectroscopy using the fluorescent dye Laurdan as a probe. Importantly, Syn DLP only very weakly interacted with pure (net uncharged) DOPC membranes, which were used as a control (Fig. 5a ). Fig. 5: Membrane interaction of Syn DLP. a Fluorescence spectroscopy using Laurdan as a fluorescent probe. LUVs were prepared with 50% DOPC and 50% of the indicated TM lipid ( w / w ) mixed with Laurdan at a 1:500 molar ratio. Laurdan fluorescence emission was measured after 30 min incubation of Syn DLP and LUVs and the ΔGP value was calculated from the spectra. Mean of three independent experiments (single measurements shown as circles) and error bars (S.D.) are shown. ns = not significant ( P > 0.05), * P < 0.05, ** P < 0.01, *** P < 0.001 based on a two-sided unpaired Student’s t-test. The ΔGP values of MGDG ( P = 0.52), SQDG ( P = 0.055), DOPG ( P = 0.00028) or DGDG ( P = 0.14) are compared to DOPC. Arrow indicates increasing membrane interaction. b LUVs were prepared with different DOPG/DOPC molar ratios (Laurdan added at a 1:500 molar ratio). Laurdan fluorescence spectra were recorded after 30 min and ΔGP values (black) were determined from the spectra. Mean of independent measurements ( n = 4) and error bars (S.D.) are shown. Arrow indicates increasing membrane interaction. c Progression of the surface pressure (black) measured over time in parallel to the SFG intensity shown in ( d ). SFG spectroscopy of 0.5 µM Syn DLP was carried out on a DMPG monolayer under reaction buffer conditions (without DTT). t = 0 s corresponds to the moment of Syn DLP addition. Mean of three independent measurements and error bars (S.D.) are shown. d The SFG spectrum in the amide I region of the DMPG monolayer (black) and after Syn DLP addition and equilibration (red) is shown. A fit of the amide I band is displayed as a line. The mean of three independent measurements is shown. SFG intensity was normalized (0–1) for better comparison. Full size image When Syn DLP was incubated with large unilamellar vesicles (LUVs) containing 50% of DOPC plus 50% of a respective TM lipid, only little membrane interaction was observed in MGDG- or DGDG-containing membranes, whereas a significant increase of the ΔGP was observed when membranes contained SQDG or DOPG (Fig. 5a ). As these two lipids carry negatively charged headgroups, Syn DLP-membrane interaction appears to contain a strong electrostatic contribution. Consequently, when Syn DLP binding to DOPG-containing membranes was analyzed using DOPC membranes with increasing DOPG mole fractions, an increasing interaction of Syn DLP with membranes was observed (Fig. 5b ). Based on these observations, all following experiments investigating the interaction of Syn DLP with membranes were always conducted with PG-containing membranes. In the here solved Syn DLP structure, we recognized two putative MIDs at the tip of the stalk based either on the quaternary (Fig. 1h , Supplementary Fig. 14a ) or the tertiary structure (Supplementary Fig. 14b ). However, when these regions were mutated, the isolated recombinant proteins still interacted with DOPG containing LUVs similar to Syn DLP wt (Supplementary Fig. 14c+d ), and thus these regions (alone) are not responsible for membrane binding of Syn DLP. Potentially, either other regions of the protein or a larger area involving multiple Syn DLP parts are responsible for membrane interaction. To obtain structural information about Syn DLPs behavior at the lipid-buffer interfaces, we next used sum frequency generation (SFG) spectroscopy to probe Syn DLP while binding a DMPG lipid monolayer. An SFG spectrum provides information about the interfacial folding and orientation of proteins. The selection rules of SFG dictate that any signal is exclusively generated by proteins bound to the interface while molecules in solution will not contribute [57] . Measurements were done in a Langmuir trough at a DMPG monolayer, in which the surface pressure was simultaneously monitored [58] . After spreading a DMPG monolayer onto the reaction buffer, an SFG spectrum was recorded at a constant surface pressure of 15 mN/m (Fig. 5c, d ). Yet, the surface pressure significantly increased from 15 to ~26 mN/m upon Syn DLP addition (Fig. 5c ), indicating Syn DLP binding to and intercalating into the membrane, resulting in lipid reassembly. When the pure DMPG layer was analyzed via SFG, a resonance signal in the amid I region at around 1738 cm −1 arose due to characteristic carbonyl stretch vibrations of the lipid headgroups (Fig. 5d , black). After injection of Syn DLP into the subphase of the trough, a broad amide I band (~1625 to ~1700 cm −1 ) was observed, originating from protein backbone vibrations (Fig. 5d , red), which indicated highly ordered binding of Syn DLP at the lipid monolayer [57] . The data were fitted using methods outlined previously [59] . The spectra were dominated by a feature at 1654 cm −1 , which is assigned to α-helical structures. Significantly weaker side bands centered at 1633 and 1680 cm −1 are assigned to β-strands structure. The dominance of α-helical SFG signal demonstrated that the structure observed via CD and cryo-EM for the solution state is maintained when Syn DLP binds to DMPG lipid interfaces. Interestingly, the resonance near 1738 cm −1 related to the PG carbonyl group remained largely unchanged after Syn DLP binding, indicating the lipid head groups remained ordered when interacting with the protein. This supported the assumption of charge interactions involved in the binding mechanism, since such interactions will align the lipid headgroups in the process. To investigate the interactions of Syn DLP with the lipid acyl chains, we recorded SFG spectra in the C–D stretching range using lipids with perdeuterated acyl chains. The deuteration allows monitoring the state of the lipid layer without interference by protein C–H modes. The spectra (Supplementary Fig. 15 ) showed a signal increase for the acyl CD 3 modes, which strongly suggested the acyl chains became more ordered with Syn DLP binding, which could be the result of the ordering effect of charge-charge interactions between protein and lipid interface or intercalation of protein side chains into the lipid layer. To glean information about the assembly process of Syn DLP on lipid surfaces, we have recorded amide spectra as a function of time (Supplementary Fig. 16 ). While the spectral shape of the protein amide I band centered around 1653 cm −1 was very similar for the interaction time, the intensity grew and then remained constant after 1500 s. The surface tension data showed that binding began to saturate after ca. 250 s. The SFG amplitude, which is sensitive to both the number of proteins and also the orientational order, increased on a similar timescale. While protein assembly often takes place in two steps—fast binding followed by a slower assembly process, the observation that the SFG signal was not lacking behind the surface tension kinetics indicated that Syn DLP swiftly formed an ordered layer after lipid binding. The secondary and tertiary structures remained stable throughout the assembly process since the spectral shape of the amide I band did not change significantly. This indicated that Syn DLP binds as a stable, folded unit which then quickly assembled into its final binding pose. As lipid-stimulation of the GTPase activity is a characteristic feature of many (eukaryotic) DLPs [18] , we investigated the interplay between Syn DLP, PG lipids and GTP. SFG spectra of Syn DLP bound to a DMPG monolayer with GTP present in solution (Supplementary Fig. 17 ) showed that, while the overall amide I signal was somewhat lower than what has been observed without GTP, the spectral shape remained unchanged. Ostensibly, the conformation of Syn DLP did not respond strongly to the presence of GTP. We then determined the Syn DLP GTPase activity in the presence of DOPG LUVs (Fig. 6 ). Yet, unlike many other DLPs, the GTPase activity of Syn DLP was not stimulated by membrane binding. As the inclusion of 5 mM MgCl 2 in the GTPase assay might lead to clustering of the lipid head groups and, thus, prevent lipid-stimulated GTPase activity, a measurement was additionally performed in the presence of only 0.5 mM MgCl 2 ± DOPG LUVs (Supplementary Fig. 11d ). Under these conditions, the GTPase activity in the presence of liposomes was slightly increased. Yet, the extent is not comparable to lipid-stimulated GTPase activity observed, e.g., for dynamin [30] . Fig. 6: Lipid-stimulation of the Syn DLP GTPase activity. Syn DLP GTPase activities in the presence and absence of LUVs were determined in a continuous, regenerative, coupled assay. Comparison of Syn DLP under standard measurement conditions (black) and with 50 µM DOPG LUVs (dissolved in reaction buffer, extrusion to 100 nm) added with the assay components (red). Mean of independent experiments ( n = 3) and error bars (S.D.) are shown. Data points were fitted using the Michaelis-Menten equation (Eq. ( 2 )). Fit curves are shown as lines. Full size image Syn DLP remodels membranes in vitro Finally, we tested a putative membrane remodeling activity of Syn DLP. While, in several cases, the formation of membrane tubes has been observed upon the addition of a DLP to lipids, we did not yet succeed in observing the formation of such structures. However, TM-mimicking LUVs were incubated with Syn DLP and their size distribution was analyzed via dynamic light scattering (DLS) and compared to protein and LUVs alone (Fig. 7a ). The LUVs were extruded to 100 nm and showed a signal at the expected size (Fig. 7a , black). Syn DLP alone showed two broad peaks suggesting fractions of smaller and larger assemblies (Fig. 7a , red). Yet, the mixture of protein and LUVs showed a prominent peak at higher sizes, indicating the formation of protein-LUV-complexes with fused and/or clustered liposomes. Based on this information, Syn DLP-triggered membrane fusion was next analyzed with a FRET-based assay using fluorescently labeled MGDG/DOPG LUVs. Fusion of labeled and unlabeled LUVs resulted in an increasing donor fluorescence, since the FRET donor and acceptor are diluted. As simple liposome tethering is not expected to significantly alter the mean distance between the FRET donor and acceptor, this measurement allowed monitoring the kinetics of membrane fusion events. IM30 of Synechocystis sp. PCC 6803, a protein with a pronounced fusogenic activity [60] , was used as a positive control (Supplementary Fig. 18 ). When isolated Syn DLP wt was mixed with labeled LUVs, the donor fluorescence increased over time, and the increase in donor fluorescence strongly depended on the Syn DLP concentration (Fig. 7b, c ). Conclusively, we observed a potential fusion activity of Syn DLP, as has been observed previously also for other BDLPs [42] , [43] , [61] . The two investigated mutants Syn DLP C777A and Syn DLP HPRN-AAAA also showed an increased donor fluorescence, yet in case of the assembly-defect Syn DLP HPRN-AAAA mutant with a lower efficiency (Supplementary Fig. 19 ). Interestingly, the addition of GTP had no impact on the fusogenic activity of Syn DLP wt (Supplementary Fig. 20 ). Noteworthy, the here observed membrane fusion activity of Syn DLP might, in the end, indicate a membrane destabilizing activity, which results in liposome fusion in vitro. The exact membrane activity of Syn DLP will be analyzed with complementing methods in future experiments. Fig. 7: Membrane fusion activity of Syn DLP. a Size distribution of protein and LUVs was analyzed using DLS and relative intensities of the respective sizes are shown. MGDG/DOPG (60%/40%, w / w ) LUVs (black), Syn DLP (red) or a mixture of LUVs and Syn DLP (blue) were incubated in reaction buffer and measured. From each condition the size distribution of three independent measurements (+ three technical replicates of each measurement) are shown. b Fusion of MGDG/DOPG (60%/40%, w / w ) LUVs was measured in the presence of increasing Syn DLP concentrations using a FRET-based fusion assay. Curves showing the donor fluorescence over the first 100 s after mixing LUVs with protein. The relative fusion activities were calculated as described in the methods section. The curves represent the mean of three independent measurements. The whole measurement as well as the positive control containing 2 µM of the fusogenic protein IM30 are shown in Supplementary Fig. 18 . c Initial fusion rates (black) were calculated from the curves in ( b ) defined as the slope of a linear regression of the first 20 s. Mean of independent measurements ( n = 3) and error bars (S.D.) are shown. Full size image Biogenesis, maintenance and dynamic rearrangement of cyanobacterial TMs are still not understood on the molecular level. In recent years, some proteins have been identified as being involved in the formation of highly curved membrane regions, in membrane fusion and/or membrane repair. One of the currently best-characterized proteins is IM30 (also known as VIPP1), a bacterial homolog of the ESCRT-III core subunit of the eukaryotic ESCRT complex [62] , [63] , [64] . In recent years, several homologs of previously assumed typical eukaryotic proteins involved in membrane dynamics have been identified in bacteria, indicating that processes, which were believed to be of eukaryotic origin, have, in fact, evolved in prokaryotes. Yet, these proteins might fulfill different functions in pro- vs . eukaryotes [65] . Cyanobacteria contain several putative genes encoding DLPs, which can be grouped into different clades depending on their genetic context. E.g., in the KGK clade of cyanobacterial DLPs typically a protein containing a KGK domain is encoded downstream of the DLP [44] . Syn DLP, a member of this clade, has recently been identified as a cyanobacterial DLP, and the involvement of Syn DLP in TM dynamics has been suggested [44] . Isolated Syn DLP forms oligomers of ~40–50 molecules in solution in the absence of nucleotides and/or membranes (Fig. 1a, b ). Nucleotide- and membrane-independent oligomerization has been reported for eukaryotic DLPs, such as dynamin [10] . However, this is a unique feature not described in the field of bacterial DLPs thus far [35] , [39] , [41] , [42] , [43] . Typically, DLPs oligomerize upon nucleotide-binding or upon binding to membrane surfaces [18] , and EM micrographs of the here observed Syn DLP oligomers (Fig. 1b ) looked, in fact, very similar to lipid-free oligomers formed by human Drp1 in the presence of GTP [50] . However, in contrast to Drp1, Syn DLP oligomers assemble already in the absence of nucleotides. Within the Syn DLP oligomer, individual monomers interact via ionic, polar and hydrophobic interactions, similar to what has been observed in other DLP assemblies [27] , [50] , [51] . Based on the Syn DLP oligomer structure, defined oligomerization interfaces can be assigned in the stalk region (Supplementary Fig. 7 ). These include interface 2, which mediates the formation of a stable dimeric unit, and interfaces 1 and 3, both critical for assembly of higher-order oligomers [27] , [51] . Noteworthy, in contrast to other BDLP structures, such as the structure of Np BDLP that is most closely related to fusion DLP s [35] , [66] , the here presented Syn DLP oligomer structure resembles a fission DLP structure, similar to classical eukaryotic dynamin or Drp1 [27] , [50] , that has not been observed in bacteria before. Detailed structural comparisons between Syn DLP and bacterial and eukaryotic DLPs demonstrate a close relationship between Syn DLP and eukaryotic representatives, indicating Syn DLP being the closest known bacterial ancestor of eukaryotic dynamin, Drps and Mx proteins (Fig. 2c , Supplementary Figs. 8 , 10 ). An intramolecular disulfide bridge, which stabilizes the BSE domain, is observed in the Syn DLP structure (Fig. 3a ). When the formation of the disulfide bridge was eliminated by replacing C777 with alanine, the resulting protein Syn DLP C777A was correctly folded and still formed oligomers, yet, its thermodynamic stability, as well as GTPase activity, were significantly reduced (Fig. 3c–g , Table 2 , Table 3 ), albeit the mutation does not directly affect the active site. This indicated an impact of the BSE domain on the Syn DLP GTPase activity. Stabilization of the BSE helix bundle via the formation of an intramolecular disulfide bridge is a concept that has not been described before, and thus far an intramolecular disulfide bridge has solely been observed in the membrane-interacting domain (paddle domain) of the eukaryotic DLP Ct Mgm1 [67] . Interestingly, the two cysteine residues involved in disulfide bridge formation in Syn DLP are conserved across the cyanobacterial KGK clade DLPs (Supplementary Fig. 21 ). Thus, it can be assumed that a disulfide bridge-stabilized BSE domain is a general feature observable in this clade of cyanobacterial DLPs. In fact, several proteins in the cyanobacterial cytoplasm contain disulfide bridges, and the (in part reversible) formation of disulfide bridges is mediated by the thioredoxin system [68] , [69] , [70] . Thus, it might even be possible that a reversible formation of the disulfide bridge in the BSE domain is involved in the regulation of the Syn DLP activity. An extended function of the BSE domain in bacterial DLPs, in general, might be indicated by the observation that all thus far resolved BDLP structures, including the Syn DLP structure described here (Fig. 1h ), show a BSE domain consisting of a four-helix bundle [35] , [39] , [41] , [43] , whereas eukaryotic DLPs typically have a three-helix bundle BSE. However, albeit Syn DLP has a four-helical BSE domain, structural alignments indicated a closer relationship to eukaryotic BSE domains (Supplementary Fig. 10 ), again underlining Syn DLPs role as the closest known bacterial ancestor of eukaryotic DLPs. For most eukaryotic DLPs, such as Dyn1, Drp1, OPA1, Vps1p, Sey1p or Mgm1p, and for BDLPs, like Np BDLP or Ms IniA, basal GTPase activities were characterized by k cat values in the range of 0.04–5 min −1 (reviewed here [21] ), which is lower than the here observed Syn DLP turnover rate of ~45 min −1 (Table 3 ). However, the GTPase activity of DLPs is often linked to their oligomeric state, and the turnover rate of many DLPs substantially increases upon oligomerization, for example, on an appropriate lipid template [18] , [21] . Mechanistically, a helical DLP polymer forms on the membrane via defined oligomerization contacts in the stalk, followed by the dimerization of GDs from adjacent rungs. This transverse GD-GD interface leads to the stabilization of critical GD residues and finally assembly-stimulated GTPase activity [22] , [71] , [72] . As mentioned earlier, Syn DLP forms stable oligomers already in the absence of nucleotides and/or membranes (Fig. 1a, b ), and putatively oligomerization stimulates its GTPase activity resulting in the measured high basal GTPase activity. Thus, it was reasonable to assume that GD interactions within the Syn DLP oligomer stabilize the enzymatic GTPase core, as observed for other DLPs [22] , [33] , [73] . Yet, the determined cryo-EM structure of Syn DLP did not indicate transverse contacts between GDs of adjacent monomers. Thus, longitudinal GD contacts within the oligomer might stimulate the Syn DLPs GTPase activity. The structure of the Syn DLP oligomers revealed only a small interface between adjacent GDs, whereas a large area of the GD of monomer 1 contacts the BSE1 domain of monomer 2 (Supplementary Figs. 8b , 22 ). The GD-BSE1 contact area is significantly expanded when compared to similar DLP assemblies [27] , [50] (Supplementary Fig. 8b ). Thus, we next analyzed the impact of these contacts on the Syn DLPs GTPase activity. A straight-forward mutational approach by substituting the respective contact residues in the GD was not possible, as the residues could not be unequivocally identified in the oligomer structure due to the intermediate resolution of the GD. While we created a mutant where eleven residues in the BSE1 (R12, N16, E20, R23, P26, S30, D33, S35, E38, G42, L45) that contact the GD were replaced, the resulting protein was prone to aggregation and not suitable for subsequent analyses. Therefore, we aimed to analyze an assembly-impaired Syn DLP variant ( Syn DLP HPRN-AAAA ) to reduce the formation of longitudinal GD-GD and BSE1-GD interactions. Isolated Syn DLP HPRN-AAAA showed lowered thermodynamic stability (Fig. 4d, e , Table 2 ) and was predominantly dimeric (Fig. 4c ). Thus, the mutant protein likely did not establish any lateral contacts to adjacent monomers anymore that involve the GD, which potentially increases the Syn DLP GTPase activity. The turnover rate of the mutant protein was reduced by ~60% compared to Syn DLP wt (Fig. 4f , Table 3 ). Thus, we propose that uncommon longitudinal interactions between GDs and interactions between the GD and the BSE1 established in the Syn DLP oligomers result in the observed high basal GTPase activity. This assumption is further supported by the observation that the disulfide bridge stabilizes the BSE domain, which affects the GTPase activity as described above. Taken together, while intramolecular GD-BSE1 interactions are described for other DLPs [27] , [52] , the Syn DLP structure and the analysis of an assembly-defective mutant indicate an additional role of the BSE domain for GTPase activation. It remains to be shown how Syn DLP oligomerization and futile GTP hydrolysis might be prevented in vivo, likely by accessory proteins. As DLPs are generally membrane-active, Syn DLP was proposed to be a peripherally membrane-attached protein. Syn DLP specifically interacts with negatively charged TM lipids (Fig. 5 ). Interaction with lipids containing a negatively charged headgroup is well-described for other DLPs, such as eukaryotic Drp1 and dynamin, as well as bacterial Bs DynA and Ms IniA [29] , [41] , [74] , [75] . A common feature of many DLPs is their ability to tubulate liposomes in vitro, which illustrates their membrane remodeling capabilities [35] , [43] , [76] , [77] . Yet, we did not succeed to observe Syn DLP-induced liposome tubulation under the tested experimental conditions. However, Syn DLP appeared to be capable of fusing liposomes in vitro in a nucleotide-independent process (Fig. 7 , Supplementary Fig. 18 ), albeit the Syn DLP oligomer structure resembles structural elements typically observed in fission DLP structures, as discussed above. The molecular mechanism of DLP-mediated membrane activity still is largely enigmatic. Yet, Syn DLP interaction with liposomes may result in membrane destabilization, a process needed for both membrane fusion as well as fission. A membrane destabilizing activity is well conceivable due to the observation that Syn DLP not only binds to but intercalates into PG containing membranes (Fig. 5c ), which induces perturbations in the lipid structure. Such a disruption of the lipid bilayer structural integrity is also proposed to play a role in atlastin-mediated membrane fusion caused by a C-terminal amphipathic helix [78] . Like Syn DLP, Bs DynA was shown to fuse membranes in absence of nucleotides, at least in vitro, and also in case of Bs DynA, liposome tubulation has not been observed thus far [42] . Recently, an involvement of Bs DynA in membrane repair after phage infection has been suggested [36] , and it appears reasonable to assume an involvement of Syn DLP in membrane repair processes caused by phage infection or other environmental stresses acting on membranes. However, phages infecting Synechocystis sp. PCC 6803 cells are not identified yet, and thus, the exact physiological activity of Syn DLP has to be analyzed in future in vivo studies. Potentially, Syn DLP is involved in the repair of membranes damaged due to the photosynthetic light reaction, e.g., via vesicle patching or budding. Also, the exact impact of GTP hydrolysis on the physiological Syn DLP function currently remains open. Looking at the structure of a Syn DLP monomer (Fig. 1h ), the connection between stalk and BSE (hinge 1) seems to be rather rigid, whereas hinge 2 consists of flexible loops with conserved proline residues (P47 and P441) known to facilitate a rotation of the BSE towards the GD [52] , [79] . The presented Syn DLP structure in the apo state shows an ‘open’ BSE conformation. A ‘closed’ BSE conformation in Syn DLP, which potentially is an intermediate in a GTP hydrolysis cycle, might be observable in structures with bound ligands. The conversion of the ‘open’ to the ‘closed’ conformation is thought to act as a power stroke in membrane remodeling processes [18] . Interestingly, the in vitro membrane activity of Syn DLP appeared to be nucleotide-independent (Fig. 7 , Supplementary Fig. 20 ). Taken together, the recently predicted cyanobacterial DLP of Synechocystis sp. PCC 6803 ( Syn DLP) is a bona fide member of the dynamin superfamily as classified by activity and structure. Syn DLP is an active GTPase that forms oligomers in solution. The Syn DLP cryo-EM structure revealed folding and oligomerization interfaces known from several eukaryotic fission DLPs in a BDLP and, thus, Syn DLP potentially represents a bacterial ancestor of eukaryotic DLPs. Furthermore, unique DLP features, such as an intramolecular disulfide bridge in the BSE domain that affected the thermodynamic stability plus the GTPase activity of Syn DLP, and an expanded intermolecular GD-BSE interface were identified in the cryo-EM structure. The presence of such GD interfaces in Syn DLP oligomers illustrates a distinctive concept for regulating the basal GTPase activity and would, thus, indicate a so far unique role of the BSE domain in a DLP. Syn DLP interacted with negatively charged TM lipids and intercalated into a DMPG monolayer. The classification of Syn DLP into fusion vs. fission DLP s is of higher complexity as it showed a membrane destabilizing activity, resulting in liposome fusion in vitro, albeit the structure of the Syn DLP oligomer resembles elements typically observed in fission DLP s. Future studies will address the exact mechanism of membrane binding and remodeling including the identification of the membrane binding site, the role of nucleotide binding and hydrolysis, and the in vivo function of Syn DLP in the cyanobacterium. Cloning, expression, and purification of Syn DLP The gene coding for Syn DLP ( slr0869 ) was amplified via PCR using genomic Synechocystis sp. PCC 6803 DNA as a template (for primers, see Supplementary Table 1 ). The NsiI/XhoI restriction digested DNA fragment was ligated into the NsiI/XhoI restriction digested vector pET303-CT/His (Thermo Fisher Scientific, Waltham, MA, USA), resulting in the plasmid pET303- slr0869- CT/His. The mutation in Syn DLP C777A and Syn DLP K61A was introduced via site-directed mutagenesis (for primers, see Supplementary Table 1 ). For expression of Syn DLP HPRN-AAAA , Syn DLP 648-665GS and Syn DLP 667-675GS the pET303- slr0869 -CT/His plasmid was mutated via Gibson assembly [80] (for primers, see Supplementary Table 1 ). For protein production, individual clones of transformed E. coli Rosetta-gami TM 2 (DE3) cells (Novagen, Darmstadt, Germany) were used to inoculate 1 L LB medium (100 µg/ml ampicillin), and cells were grown at 37 °C until an OD 600 of 0.6–0.8 was reached. Expression of Syn DLP was induced via the addition of IPTG (1 mM). Cells were grown at 20 °C overnight, harvested by centrifugation the following day, and the resulting pellet was snap frozen in liquid nitrogen and stored at −20 °C until used. The pellet was resuspended in buffer (50 mM NaH 2 PO 4 , 300 mM NaCl, 10% glycerol, 10 mM imidazole, pH 8.0) and cells were homogenized using a Potter-Elvehjem device and lyzed with a LM20 microfluidizer® (Microfluidics international cooperation, Westwood, MA, USA) for four rounds at a pressure of 18000 psi. The crude cell extract was centrifuged (15,000 × g , 10 min, 4 °C) and the supernatant was mixed with a Ni-NTA matrix (Protino®, Macherey-Nagel, Düren, Germany) equilibrated with 50 mM NaH 2 PO 4 , 300 mM NaCl, 10% glycerol, 10 mM imidazole, pH 8.0. After incubation at 4 °C for 2 h, the matrix was washed six times with the same buffer supplemented with either 20, 40, or 50 mM imidazole, respectively. Syn DLP was finally eluted with a buffer containing 500 mM imidazole. Next, Syn DLP was incubated with 20 mM DTT for half an hour at 4 °C and the protein was further purified via size exclusion chromatography using a self-packed Sephacryl S-400 HR column (Cytiva, Freiburg, Germany) equilibrated with 20 mM HEPES pH 7.4, 0.2 mM DTT on an ÄKTA purifier 10 system (GE Healthcare, Munich, Germany). Main peak fractions were collected and concentrated. Protein concentrations were determined using a reducing agent compatible BCA assay kit (Pierce TM , Thermo Fisher Scientific, Waltham, MA, USA). The purity of the protein was estimated by SDS-PAGE (calculated molecular mass of Syn DLP: 93 kDa) and the protein was typically ≥95% pure. Per liter E. coli culture, 1–2 mg protein was purified. All subsequent experiments were performed with heterologously expressed and purified protein (except the immunoprecipitation experiment in Supplementary Fig. 1 , which showed expression of native Syn DLP). DTT titration Purified Syn DLP was incubated for 15 min at RT with different DTT concentrations (final concentrations 0.1–500 mM DTT). The samples were mixed with SDS sample buffer, incubated at 95 °C for 5 min, and separated by SDS-PAGE (for the uncropped gel, see Source Data file). GTPase assay GTPase activity was measured using a modified version of a continuous, regenerative, coupled GTPase assay [81] . Reaction buffer (final concentrations: 20 mM HEPES pH 7.4, 150 mM NaCl, 7.5 mM KCl, 5 mM MgCl 2 , 0.2 mM DTT) was mixed with phosphoenolpyruvate (final concentration: 1 mM). 2.33% ( v / v ) PK/LDH (Sigma-Aldrich Chemie GmbH, Taufkirchen, Germany) and NADH (final concentration: 0.6 mM) (Carl Roth GmbH + Co. KG, Karlsruhe, Germany) were added to obtain a master mix. Different concentrations of GTP (Sigma-Aldrich Chemie GmbH, Taufkirchen, Germany) dissolved in 20 mM HEPES pH 7.4 were added to the master mix, and the solutions were incubated at 4 °C for 15 min to convert all remaining GDP to GTP. The protein (0.5 µM final concentration) and pure buffer (blank) were placed into a 96-well plate and mixed with the GTP-containing master mix, resulting in a final volume of 150 µl per well. The absorption at 340 nm was observed with a microplate reader (FLUOstar® Omega, BMG Labtech GmbH, Ortenberg, Germany) using the software Omega (version 1.3) at 30 °C over 2–3 h to make sure that even at the lower GTP concentrations all NADH was oxidized. The activities at different substrate concentrations were calculated using the MARS Data Analysis software (version 2.10 R3) and MS Excel (version 2208) as follows: The absolute value of the slope of the blank measurement was subtracted from the absolute value of the maximum linear absorption decrease at 340 nm, yielding the corrected decrease of the absorption at 340 nm over time (Δ A corr ). The GTP hydrolyzing activity was calculated with Eq. ( 1 ): 
    Activity=A_corr/d*ε*c_Protein
 (1) ε refers to the molar extinction coefficient of NADH at 340 nm (6220 M −1 cm −1 ), and d is the thickness of 150 µl sample volume in a 96-well plate (0.38 cm). The calculated activities were plotted against the GTP concentrations. The data points were fitted with a Michaelis-Menten equation (Eq. ( 2 )) using Origin TM (version 9.60) (OriginLab Corporation, Northampton, MA, USA) to determine the turnover rate ( k cat ) and the Michaelis-Menten constant ( K m ). Activity([GTP])=[GTP]*k_cat/[GTP]+K_m
 (2) Analytical size exclusion chromatography A Superose® 6 Increase 3.2/300 column (Sigma-Aldrich Chemie GmbH, Taufkirchen, Germany), equilibrated with reaction buffer, was loaded with 30 µl of a 10 µM protein solution. Proteins were eluted using an ÄKTA purifier 10 system (GE Healthcare, Munich, Germany) at 7 °C and a flow rate of 0.03 ml/min. The standard proteins thyroglobulin (669 kDa) Ferritin (440 kDa), Aldolase (158 kDa), Conalbumin (75 kDa) and Ovalbumin (44 kDa) (Sigma-Aldrich Chemie GmbH, Taufkirchen, Germany) were used for protein mass estimation. Chromatograms were recorded using the software UNICORN (version 5.10). Circular dichroism spectroscopy The CD spectrum of 1 µM protein was recorded in 10 mM HEPES, pH 7.4, using a JASCO J-1500 CD spectrometer with an MPTC-490S temperature-controlled cell holder (JASCO cooperation, Tokyo, Japan) and the software JASCO Spectra Manager (version 2.15.01). The spectral range was 200–250 nm with a scan rate of 50 nm/min, 1 mm cell length, 1 nm steps, 5 nm bandwidth, 1 s data integration time, 8-time accumulation at 20 °C. For measurements of the thermal stability, the spectra were recorded from 200 to 250 nm with a scan rate of 100 nm/min, 1 mm cell length, 1 nm steps, 5 nm bandwidth, 1 s data integration time, 1-time accumulation at increasing temperatures starting from 20 °C to 84 °C recorded in 2 °C steps and a heating rate of 1 °C/min. Each spectrum was smoothed using the Savitzky-Golay filter from the software JASCO Spectra Analysis (version 2.15.01). Three individual measurements were averaged for each sample. For this purpose, the data sets were interpolated, as the measurements were recorded at slightly different actual temperatures. The interpolated data sets were normalized and averaged, resulting in a melting curve. The transition temperature ( T m ) was determined using an adapted Boltzmann fit (Eq. ( 3 )). This fit is based on a two-state unfolding mechanism and enables linear slopes in the plateau areas of the curve: 
    θ_meas(T)=(T*m_N+θ_N)-(T*m_D+θ_D)/1+e^T-T_m/dT+(T*m_D+θ_D)
 (3) θ meas refers to the measured ellipticity at 222 nm and T is the temperature. θ N and θ D are the ellipticities at the plateau regions of the native and the denatured protein, m N and m D are the slopes of the corresponding plateaus. Data procession and the fit were performed using Origin TM (version 9.60) (OriginLab Corporation, Northampton, MA, USA). ANS fluorescence thermal shift assay Proteins were mixed with the fluorescent dye 8-anilinonaphthalene-1-sulfonic acid (ANS), which shows increased fluorescence emission when bound to hydrophobic pockets found at surfaces of folded proteins or to hydrophobic regions becoming accessible due to protein unfolding. Thus, ANS can be used to monitor protein unfolding. For an FTSA, Syn DLP (5 µM) was mixed with 50 µM of the fluorophore ANS in reaction buffer. Fluorescence emission was recorded from 400 to 600 nm using a JASCO FP-8500 fluorescence spectrometer (JASCO cooperation, Tokyo, Japan) and the software JASCO Spectra Manager (version 2.9.0.7) upon excitation at 370 nm. Integration time was 0.1 s, and the excitation and emission slits corresponded to a spectral resolution of 2.5 nm. Spectra were recorded with a scan rate of 200 nm/min, 1 nm steps at temperatures ranging from 20 to 80 °C in 1 °C steps, and a heating rate of 1 °C/min. The fluorescence intensity at 470 nm was used as a measure of the Syn DLP folding state. Three independent measurements were combined for each sample. The data sets were interpolated due to different actual temperatures and then averaged to obtain a melting curve of the protein. The transition temperature was determined using an adapted Boltzmann fit similar to Eq. ( 3 ) (Eq. ( 4 )): 
    F_meas(T)=(T*m_N+F_N)-(T*m_D+F_D)/1+e^T-T_m/dT+(T*m_D+F_D)
 (4) F meas denotes the measured fluorescence intensity at 470 nm, while T is the temperature. F N and F D are the fluorescence intensities at the plateau regions of the native and the denatured protein, m N and m D are the slopes of the corresponding plateaus. It is important to note that fitting using Eq. ( 4 ) could not be applied to the entire measured temperature range, as the ANS fluorescence strongly depends on the temperature besides binding to a folded or denatured protein. Therefore, the adjusted data included a temperature range of 20–25 °C that captured the transition phase. Data procession and the fit were performed using Origin TM (version 9.60) (OriginLab Corporation, Northampton, MA, USA). Preparation of large unilamellar vesicles The lipids DOPG (1,2-dioleoyl- sn -glycero-3-phosphoglycerol), DOPC (1,2-dioleoyl- sn -glycero-3-phosphocholine), DMPG (1,2-dimyristoyl- sn -glycero-3-phosphoglycerol), MGDG, DGDG and SQDG as well as the fluorescently labeled lipids LissRhod-PE (Lissamine Rhodamine PE; 1,2-dioleoyl- sn -glycero-3-phosphoethanolamine-N-(Lissamine Rhodamine B sulfonyl) (ammonium salt)) and NBD-PE (1,2-distearoyl- sn -glycero-3-phosphoethanolamine-N-(7-nitro-2-1,3-benzoxadiazol-4-yl)) were all purchased from Avanti Polar Lipids, Inc. (Birmingham, AL, USA). For the preparation of LUVs, the organic solvent (CHCl 3 /MeOH 2:1 ( v / v )) was evaporated under a gentle stream of nitrogen gas followed by vacuum desiccation overnight to remove any traces of solvent. The dried lipid film was hydrated in an appropriate buffer and LUVs were prepared by five cycles of freezing in liquid nitrogen and thawing at 37 °C. For the membrane fusion assay, the LUVs were extruded 15 times through a 100 nm filter (Nucleopore Track-Etch Membrane, Whatman, Sigma-Aldrich GmbH, Taufkirchen, Germany) using an extruder (Avanti Polar Lipids, Inc., Birmingham, AL, USA). Laurdan fluorescence measurements The fluorescent dye Laurdan (6-dodecanoyl- N , N -dimethyl-2-naphthylamine) incorporates into lipid bilayers. Its fluorescence emission characteristics depend on the polarity of the environment. Determining Laurdan fluorescence emission spectra can be used to monitor changes in the membrane polarity, e.g., caused by protein adhesion to a membrane surface. The effect of Syn DLP on different model membrane systems containing DOPC and varying amounts of TM lipids (MGDG, DGDG, SQDG, DOPG) was tested. Laurdan (Sigma-Aldrich Chemie GmbH, Taufkirchen, Germany) was added at a molar ratio of 1:500 to a 0.5 mM lipid solution prior to LUV formation. LUVs were prepared in 20 mM HEPES, pH 7.4 as described above. 0.1 mM LUVs were incubated with 0.5 µM Syn DLP in 20 mM HEPES pH 7.4 for 30 min at 25 °C. Laurdan fluorescence emission spectra were measured at 25 °C from 400 to 550 nm using a Fluoromax-4 spectrometer (Horiba Scientific, Kyoto, Japan) and the software FluorEssence (version 3.8) with excitation at 350 nm. The excitation and emission slit widths corresponded to a spectral resolution of 3 nm. The data were further analyzed using MS Excel (version 2208) and Origin TM (version 9.60) (OriginLab Corporation, Northampton, MA, USA). Spectral changes were quantified using the Generalized Polarization (GP) value [82] , which was calculated for each spectrum (Eq. ( 5 )): 
    GP=I_440-I_490/I_440+I_490
 (5) Here, I 440 and I 490 are the Laurdan fluorescence emission intensities at 440 and 490 nm, respectively. ΔGP values were obtained by subtraction of the GP value of LUVs without protein. SFG spectroscopy SFG spectroscopy was used to obtain selective information about the orientation and conformation of Syn DLP at membrane-buffer interfaces. For a more detailed description of this method concerning interfacial protein structure elucidation, see, for example, [57] , [83] , [84] , [85] . All SFG experiments were performed according to established procedures [59] , [86] using SFGTools ( https://github.com/james-d-pickering/SFGTools ) and Matlab (version 2022a). Briefly, two laser beams (one visible and one tunable laser) overlap at the sample to generate light at their sum-frequency (ω VIS + ω IR = ω SFG ). Pulses were provided by a Ti:sapphire laser (Mai Tai, Spectra-Physic, Santa Clara, CA, USA), amplified (Spitfire Ace, Santa Clara, CA, USA) and pumped (Nd:YLF laser, Empower, Spectra-Physics, Santa Clara, CA, USA). The resulting beam had a pulse repetition rate of 1 kHz and a duration of about 40 fs. The power was about 5 mJ at 800 nm. One part of the beam was used to generate the IR beam in an optical parametric amplifier (TOPAS, Light Conversion, Vilnius, Lithuania). The SFG signal was detected by an EMCCD camera (Newton, Andor, Belfast, Northern Ireland). All spectra were recorded in the polarization setting ssp (s-SFG, s-VIS, and p-IR) and averaged for 600 s, respectively. For further spectral analysis, the background was subtracted, and the spectra were normalized using a non-resonant reference spectrum (gold-coated silicon wafer). The spectra were fitted assuming a Lorentzian line shape and using the software Origin TM (version 9.60) (OriginLab Corporation, Northampton, MA, USA). Dynamic light scattering (DLS) Size distributions of proteins and LUVs were determined via DLS. MGDG/DOPG (60%/40%, w / w ) LUVs were prepared in 20 mM HEPES pH 7.4, 0.2 mM DTT and extruded to 100 nm, as described above. Either 1 µM Syn DLP, 0.1 mM LUVs or a mixture of both were incubated at RT in reaction buffer for 15 min and measured in a Zetasizer Pro (Malvern Panalytical Ltd, Malvern, UK) using the software ZS Xplorer (Version 2.3.1.4) at 25 °C using backscatter. After an equilibration time of 60 s, three individual samples were measured three times and analyzed via the manufacture’s software, finally yielding in intensity-weighted size distribution. Membrane fusion assay Membrane activity of Syn DLP was tested using a FRET (Förster resonance energy transfer)-based LUV fusion assay, as described in detail recently [60] , [87] . Unlabeled MGDG/DOPG (60%/40%, w / w ) LUVs and labeled LUVs, containing 0.8 mol% of the FRET dyes LissRhod-PE and NBD-PE each, were prepared in 20 mM HEPES pH 7.4, 0.2 mM DTT, as described. Unlabeled and labeled LUVs were mixed at a ratio of 9:1 ( v / v ), and when the two LUV species fused, the FRET dyes redistributed over the membrane leading to decreased FRET and increased donor emission. Mock fused LUVs, containing solely 1/10 of the fluorescently labeled lipids, were produced and measured to correct for bleaching. Protein solutions were incubated in reaction buffer at 25 °C 10 min prior to the measurement. After that, the solution containing Syn DLP in different concentrations (0–5 µM) and the mixture of unlabeled and labeled LUVs (final concentration: 0.1 mM) were rapidly mixed, and the measurement was started immediately. The fluorescence emission of the FRET donor NBD-PE was monitored at 535 nm for 15 min at 25 °C after excitation at 460 nm using a Fluoromax-4 spectrometer (Horiba Scientific, Kyoto, Japan) and the software FluorEssence (version 3.8). The slit widths for excitation and emission corresponded to a spectral resolution of 2 and 10 nm, respectively. The fusion activity of 2 µM of the cyanobacterial IM30 protein, which is well-known to trigger the fusion of membranes containing TM lipids [60] , [88] , [89] , [90] , was measured as a positive control. The data were further analyzed using MS Excel (version 2208) and Origin TM (version 9.60) (OriginLab Corporation, Northampton, MA, USA). Relative fusion activities were calculated via conversion of the raw fluorescence data by Eq. ( 6 ): 
    Fusion activity (t)=I-I_0/I_M-I_0
 (6) Here, I 0 is the NBD-PE fluorescence intensity of the negative control measured without protein, I M is the intensity of the mock fused LUVs and I the measured sample at every point in time t . The initial fusion rates were determined by the slope of linear regression of the first 20 s of every fusion curve. Negative staining electron microscopy For negative-staining electron microscopy, 3.5 µl of the sample was applied to glow-discharged (PELCO easiGlow Glow Discharger, Ted Pella Inc., Redding, CA, USA) continuous carbon grids (Cu 300 hex grids; Electron Microscopy Sciences, Hatfield, PA, USA; in-house coated with carbon film). The sample was incubated on the grid for 1 min. Then the grid was side-blotted using filter paper, washed with 3.5 µl water, stained with 3.5 µl 2% uranyl acetate for 30 s, and air-dried. The grids were imaged with a 120 kV Talos L120C electron microscope (Thermo Fisher Scientific, Waltham, MA, USA; FEI Company, Hillsboro, OR, USA) equipped with a CETA camera at a pixel size of 4.05 Å/pixel (36 kx magnification) at a nominal defocus of 1.0–2.5 µm. Cryo-electron microscopy (cryo-EM) and image processing Syn DLP samples were prepared by applying 3.5 µl Syn DLP (~3.0 mg/mL in 5 mM MgCl 2 , 7.5 mM KCl, 20 mM HEPES pH 7.4) to glow-discharged (PELCO easiGlow Glow Discharger, Ted Pella Inc., Redding, CA, USA) Quantifoil grids (R1.2/1.3 Cu 200 mesh; Electron Microscopy Sciences, Hatfield, PA, USA). The grids were plunge-frozen in liquid ethane using a Thermo Fisher Scientific Vitrobot Mark IV (Thermo Fisher Scientific, Waltham, MA, USA) set to 90% humidity at 20 °C (blotting force −10, blotting time 3 s). A total of 8322 micrographs were recorded on a 200 kV Talos Arctica G2 (Thermo Fisher Scientific, Waltham, MA, USA) electron microscope equipped with a Bioquantum K3 (Gatan, Inc., Pleasanton, CA, USA; controlled by Digital Micrograph (version 3.32.2403.0)) detector operated by EPU (version 2.11.0.2368REL) and TIA (version 5.0.0.2896) together with FluCam viewer (version 6.15.3.22415) (Thermo Fisher Scientific, Waltham, MA, USA). Micrographs were collected as 30-frame movies in super-resolution mode at 0.8685 Å/pixel and a cumulative dose of 26.5 e − /Å 2 and a nominal underfocus of 2.0–4.0 μm. Movie frames were gain-corrected, dose weighted, and aligned in super-resolution using cryoSPARC Live [91] (version 3.2). Initial 2D classes were produced using the auto picker implemented in cryoSPARC Live. All the following image processing steps were performed using cryoSPARC (version 3.2). The 7 best-looking classes were used as templates for the template picker. The resulting 10,000,000 particles were extracted with 450 px box size (Fourier cropped to 256 px) and subjected to multiple rounds of 2D classification. The cleaned particle set contained 2,685,000 particles. The particles were further divided by ab initio reconstruction into two classes. The first class contained 1,806,000 particles and was used for further processing. The ab initio model of the first class was further refined using multiple rounds of non-uniform refinement and hetero-refinement with imposed C2 symmetry. Finally, the particles were reextracted to the full resolution (super-resolution) and subjected to non-uniform refinement (including group and per-particle CTF refinement), followed by local refinement. The final reconstruction was determined to have a global resolution of 3.7 Å (auto-masked, FSC = 0.143) and was based on 977,200 particles. Local filtering and determination of the local resolution was performed using cryoSPARC. Cryo-EM map interpretation and model building The 3D reconstruction was B-factor sharpened (B = −184.9 Å 2 ) in cryoSPARC. The handedness of the final map was determined by rigid-body fitting the BSE-domain of Np BDLP [35] into the final map using ChimeraX [92] (version 1.2.5). The locally filtered map was used for de novo model building of the BSE-domain in Coot [93] (version 0.95). The resolution in the periphery of the map did not allow model building of the GD. Thus, a model of the GD (aa 48–423) was generated using AlphaFold2 [94] , [95] . To integrate the AlphaFold2 model with the de novo model, an overlap of 40 aa at the N and C-terminus of the GD was included in the model. The AlphaFold2 model was flexibly MDFF fitted to the 3D reconstruction using ISOLDE [96] (version 1.2) and fused to the de novo model. The resulting monomer model includes aa 1–793. The monomer model was manually refined using Coot and ISOLDE before rigid body extending a total of 8 monomers to fill the complete 3D reconstruction. Non-crystallographic symmetry (NCS) parameters for the octamer were obtained by phenix.find_ncs (Phenix version 1.18). The octamer model was subjected to two cycles of auto-refinement with phenix.real_space_refine [97] (with NCS constraints and NCS refinement) and local map sharpening using LocSCALE [98] (version 0.1). After final inspection, the model was validated in phenix.validatiopn_cryoem [99] /Molprobity [100] . Reporting summary Further information on research design is available in the Nature Portfolio Reporting Summary linked to this article.